Enhancing adult nerve regeneration through the knockdown of retinoblastoma protein Tumour suppressor pathways may offer novel targets capable of altering the plasticity of post-mitotic adult neurons. Here we describe a role for the retinoblastoma (Rb) protein, widely expressed in adult sensory neurons and their axons, during regeneration. In adult sensory neurons, Rb short interfering RNA (siRNA) knockdown or Rb1 deletion in vitro enhances neurite outgrowth and branching. Plasticity is achieved in part through upregulation of neuronal PPARυ; its antagonism inhibits Rb siRNA plasticity, whereas a PPARυ agonist increases growth. In an in vivo regenerative paradigm following complete peripheral nerve trunk transection, direct delivery of Rb siRNA prompts increased outgrowth of axons from proximal stumps and entrains Schwann cells to accompany them for greater distances. Similarly, Rb siRNA delivery following a nerve crush improves behavioural indices of motor and sensory recovery in mice. The overall findings indicate that inhibition of tumour suppressor molecules has a role to play in promoting adult neuron regeneration. Recovery from neurological injury or disease frequently requires axon regrowth, a process that can be remarkably restrained and delayed in both central and peripheral neurons [1] . Less often appreciated are the considerable and persistent deficits that follow lesions of major peripheral nerve trunks, especially transection. Despite ideas otherwise, large proximal nerve lesions are associated with very poor functional recovery, rendering severe and permanent disability. Peripheral nerve injuries exceed those of the spinal cord by at least one magnitude; a complete axonal lesion at the level of the proximal sciatic nerve or brachial plexus is unlikely to be associated with the recovery of foot or hand function, respectively [2] , [3] , [4] . As might be expected from such poor outcomes, regrowth of axons across transection gaps, common forms of injury, is highly constrained and limited. Indeed, only 10% of axons from the proximal stump may eventually successfully navigate to their targets [5] . Reluctant regrowth of axons may be partially responsive to neuronal and pleiotropic growth factors, depending on their receptor expression. Some of these factors are already present at injury sites. Alternatively, intrinsic mechanisms that brake more robust outgrowth paradoxically exist within neurons, a role that likely ensures stability of complex connections in adults. After injury, the ongoing expression of these molecular ‘brakes’ attenuates regrowth. Examples include RhoA GTPase and PTEN [6] , [7] . A related issue is that signalling pathways influencing overall axon outgrowth and neuron plasticity overlap with those associated with protection and survival. Two examples include PI3K-Akt signalling downstream of many growth factors that supports both neuronal survival and axon outgrowth and HSP27, a molecular chaperone that similarly protects neurons and enhances regeneration [8] , [9] . ‘Brake’ or plasticity molecules in neurons also overlap with those that influence tumour growth; especially recognized are PTEN and PI3K. It is thus plausible that other molecules and pathways capable of altering tumour growth and that are normally expressed in stable adult neurons might offer new avenues for manipulating neurological regenerative growth. In this work we identify a classical tumour suppressor pathway involving the protein retinoblastoma (Rb) as a regulator of peripheral nerve regeneration. Rb offers opportunities to promote growth through promiscuous interactions involving a number of signalling networks that are involved in growth stimulation and have an impact on survival and apoptosis [10] . Importantly, these networks suggest that Rb might operate downstream of the canonical survival pathways of Raf-MEK and PI3K-Akt. Not previously explored in the adult nervous system, we show that Rb is widely expressed and operates to suppress neuronal plasticity. Its knockdown is associated with enhanced plasticity that translates into a robust action on local axons and their accompanying Schwann cells (SCs) during regrowth from complete nerve trunk transection. The overall findings highlight the possibilities that manipulation of tumour suppressor pathways, not routinely considered in post-mitotic neurons, might be used to enhance adult nervous system regeneration. Adult sensory neurons express the Rb protein A role for the Rb protein, a key inhibitor of cell cycle progression, commonly deleted in human tumours, has not been described in the adult nervous system. During development, Rb may have critical roles in neuronal precursor cell proliferation and neuron migration; however, it has been uncertain whether Rb expression persists within or has an impact on adult neurons [11] . Given these uncertainties, we observed its expression in a large proportion of dorsal root ganglion (DRG) sensory neurons, colabelling with neurofilament expressing large calibre neurons but also present in neurofilament-poor smaller calibre neurons ( Fig. 1 ). These patterns of expression suggested the possibility of a widespread functional role. Expression was largely neuronal within the cytoplasm and prominently displayed in nuclei. In peripheral nerve trunks, Rb was expressed almost exclusively in axons, colabelling with a neurofilament label but with relatively minor colabelling of SCs ( Fig. 2 ). Following injury, Rb was robustly expressed in axons at the injury site. SCs at the regenerative nerve front were not prominently labelled ( Fig. 2 ). S100β SC profiles surrounded the axonal Rb profiles. Distal to the site of injury, Rb was identified in profiles undergoing axonal degeneration, indicating its presence in phagocytic SCs and macrophages. After injury, Rb expression in DRG sensory neurons and in axons persisted, although there was a relative decline in its mRNA and protein levels ( Fig. 1 ; Supplementary Figs 1 and 2 ). Overall, the findings supported the possibility that Rb was poised to influence neuronal behaviour after injury. 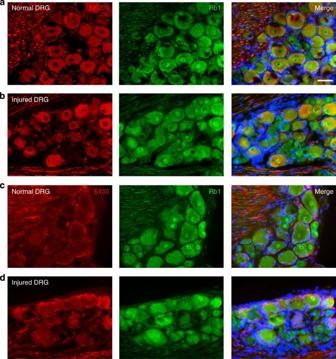Figure 1: Rb1 is expressed in sensory DRG. Transverse sections of normal adult DRG with co-expression in neurons of NF200 and Rb1, the latter in the cytoplasm and nuclei (a). Transverse section of 3d injured DRG with co-expression of NF200 and Rb1 (b). There is relatively little co-expression of Rb1 and S100β, a marker of Schwann cells, in DRG (c); As inc, following 3d axotomy injury (d). Bars=50 μm. Figure 1: Rb1 is expressed in sensory DRG. Transverse sections of normal adult DRG with co-expression in neurons of NF200 and Rb1, the latter in the cytoplasm and nuclei ( a ). Transverse section of 3d injured DRG with co-expression of NF200 and Rb1 ( b ). There is relatively little co-expression of Rb1 and S100β, a marker of Schwann cells, in DRG ( c ); As in c , following 3d axotomy injury ( d ). Bars=50 μm. 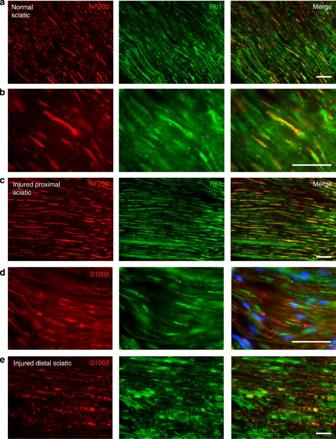Figure 2: Rb1 is preferentially expressed in neurons and axons. Expression of Rb1 in normal sciatic nerve (a). Note the colabelling with a neurofilament marker indicating expression in axons. Expression at higher power (b). Longitudinal section of 3d injured sciatic nerve proximal to the injury zone, with intense co-expression of Rb1 in NF200 labelled axons (c). Lack of co-expression of S100β and Rb1 in the proximal tip of injured sciatic nerve (d). Note that the SC S100β surrounds the Rb1 axon profiles. Limited co-expression of S100β and Rb1 in the distal segment of injured sciatic nerve, largely involving axons undergoing axonal degeneration (e). Bars=50 μm. Full size image Figure 2: Rb1 is preferentially expressed in neurons and axons. Expression of Rb1 in normal sciatic nerve ( a ). Note the colabelling with a neurofilament marker indicating expression in axons. Expression at higher power ( b ). Longitudinal section of 3d injured sciatic nerve proximal to the injury zone, with intense co-expression of Rb1 in NF200 labelled axons ( c ). Lack of co-expression of S100β and Rb1 in the proximal tip of injured sciatic nerve ( d ). Note that the SC S100β surrounds the Rb1 axon profiles. Limited co-expression of S100β and Rb1 in the distal segment of injured sciatic nerve, largely involving axons undergoing axonal degeneration ( e ). Bars=50 μm. Full size image Rb protein knockdown enhances neuron plasticity To address the potential impact of Rb expression on adult sensory neurons, we analysed their outgrowth patterns in response to Rb knockdown. This approach has predicted in vivo behaviour in response to several plasticity signals studied in previous work including RHOA and PTEN inhibition [6] , [7] . Since Rb−/− mice are embryonically lethal, suitable adult populations of their neurons are not available. Similarly, the phenotype of Rb+/− mice is highly impaired and abnormal, limiting the health and viability of their neurons [13] . In view of these concerns, as well as our intent to temporarily and locally knockdown an oncogenic molecule, we examined the impact of transient knockdown on Rb using siRNA directed specifically to neurons. First, we examined adult sensory neurons in dissociated cell culture using a lipid transfection protocol that achieves robust and predictable mRNA knockdown. We confirmed that two specific but differing Rb siRNA constructs were extensively taken up by neurons and suppressed their Rb mRNA and protein ( Fig. 3 ). No impact of scrambled sequence control siRNA was identified. Pre-injured adult sensory neurons, with an already enhanced baseline growth rate, and designed to mimic responses to in vivo injury, were exposed to Rb or scrambled siRNA for 18–20 h. Their pattern of neurite outgrowth was analysed. Rb-suppressed neurons with siRNA uptake showed an overall increase of over 50% in neurite outgrowth and maximum process length. In addition, there was a 60% rise in numbers of neurite branches ( Fig. 3e–h ). Neurons that exhibited increased plasticity were specifically those that acquired the labelled Rb siRNA construct ( Fig. 3i,j ). The findings identified an added impact of Rb suppression that was superimposed on ‘preconditioned’ accelerated outgrowth of pre-injured adult neurons. To identify whether the Rb1 siRNA knockdown strategy had an impact on growth in a separate rodent species of adult sensory neuron, we repeated the analysis in uninjured DRG neurons of adult mice exposed to Rb1 siRNA or scrambled controls. The approach similarly identified a robust impact on neurite outgrowth and branching ( Supplementary Fig. 3 ). The addition of siRNA to E2F1, a critical target of Rb, eliminated the impact of Rb1 siRNA on outgrowth and branching in rat DRG neurons, indicating a role for E2F1 in neuronal plasticity ( Supplementary Fig. 4 ). Taken together, these findings indicated a robust role for Rb in suppressing neurite outgrowth, reversed by local knockdown. 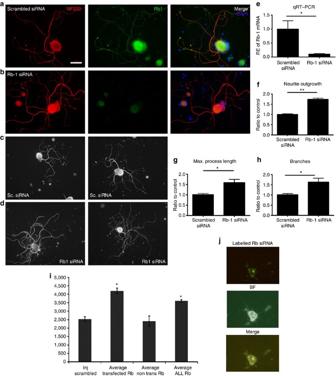Figure 3: siRNA knockdown of Rb1 increases DRG neurite outgrowth. Rb1 is co-expressed with NF200 in injured and dissociated adult DRG neurons (a). Knockdown of Rb1 with an siRNA decreases Rb1 expression (b). Images of DRG neurons with scrambled siRNA (c). Images of DRG neurons with Rb1 siRNA—note the increase in neurite outgrowth (d). (Bar=50 μm). Rb1 siRNA significantly decreases Rb1 mRNA (*P<0.001,n=4; unpaired two-tailed Student’st-test) (e). Neurite outgrowth quantified from MetaXpress, represented as a ratio in transfected neurons to control (Scrambled: 2,486±80 μm, Rb1: 4,310±114 μm, **P<0.0001,n=5; unpaired two-tailed Student’st-test) (f). Maximum process length (Scrambled: 1,258±71 μm, Rb1: 1,970±140 μm, *P<0.01,n=5; unpaired two-tailed Student’st-test) (g). Number of branches (Scrambled: 100±6, Rb1: 160±12, *P<0.05,n=5; unpaired two-tailed Student’st-test) (h). Values are means±s.e.m. Quantitation of total neurite outgrowth analysed in sensory neurons in which labelled Rb1 siRNA was specifically identified within the neuron or in all sensory neurons exposed in the culture dish to Rb1 siRNA (i). Note that enhanced neurite outgrowth is specifically associated with neurons in which visualization of labelled siRNA uptake was confirmed (scrambled versus average transfected, or average ALL Rb *P<0.0001; unpaired two-tailed Student’st-test). Labelled siRNA within harvested dissociated adult sensory neurons identified by brightfield (BF) and fluorescence (j). Figure 3: siRNA knockdown of Rb1 increases DRG neurite outgrowth. Rb1 is co-expressed with NF200 in injured and dissociated adult DRG neurons ( a ). Knockdown of Rb1 with an siRNA decreases Rb1 expression ( b ). Images of DRG neurons with scrambled siRNA ( c ). Images of DRG neurons with Rb1 siRNA—note the increase in neurite outgrowth ( d ). (Bar=50 μm). Rb1 siRNA significantly decreases Rb1 mRNA (* P <0.001, n =4; unpaired two-tailed Student’s t -test) ( e ). Neurite outgrowth quantified from MetaXpress, represented as a ratio in transfected neurons to control (Scrambled: 2,486±80 μm, Rb1: 4,310±114 μm, ** P <0.0001, n =5; unpaired two-tailed Student’s t -test) ( f ). Maximum process length (Scrambled: 1,258±71 μm, Rb1: 1,970±140 μm, * P <0.01, n =5; unpaired two-tailed Student’s t -test) ( g ). Number of branches (Scrambled: 100±6, Rb1: 160±12, * P <0.05, n =5; unpaired two-tailed Student’s t -test) ( h ). Values are means±s.e.m. Quantitation of total neurite outgrowth analysed in sensory neurons in which labelled Rb1 siRNA was specifically identified within the neuron or in all sensory neurons exposed in the culture dish to Rb1 siRNA ( i ). Note that enhanced neurite outgrowth is specifically associated with neurons in which visualization of labelled siRNA uptake was confirmed (scrambled versus average transfected, or average ALL Rb * P <0.0001; unpaired two-tailed Student’s t -test). Labelled siRNA within harvested dissociated adult sensory neurons identified by brightfield (BF) and fluorescence ( j ). Full size image As a further validation of the impact of Rb knockdown on the plasticity of sensory neurons, we harvested lumbar and thoracic DRG neurons from adult Rb1-floxed mice (FVB; 129- Rb1 tm2Brn ) and transfected them with control adenovirus (Ad-GFP (green-fluorescent protein)) or Cre recombinase expressing adenovirus (Ad-CMV (cytomegalovirus)-Cre) particles. In separate experiments the cells were infected with Ad-GFP-2A-iCre particles, which express both Cre recombinase and GFP. Neurons transfected with Ad-GFP-2A-iCre are illustrated in Fig. 4 . Rb knockdown was confirmed using qRT–PCR. As above, the patterns of neurite outgrowth were compared between neurons with Rb1 knockdown and those exposed to virus without Cre recombinase. Neurons with Rb knockdown had robust rises in neurite outgrowth, maximum process length, numbers of processes and numbers of branches ( Fig. 4 ; Supplementary Fig. 4 ). 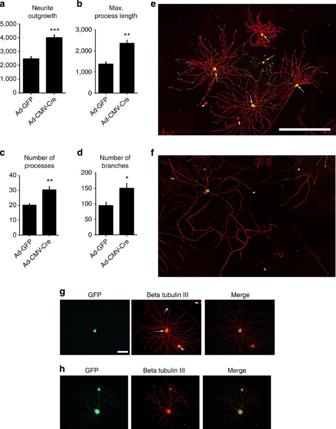Figure 4: Conditional knockdown of Rb1 in adult sensory neurons from Rb1-floxed mice is associated with enhanced neurite outgrowth. Conditional knockdown of Rb1 is associated with rises in neurite outgrowth, maximum process length, numbers of processes (neurites) and numbers of branches (a–d) (***P<0.001 fora, **P=0.001 forb, **P<0.01 forc, *P<0.05 ford;n=6/group; unpaired two-tailed Student’st-tests). Values are means±s.e.m. Low-power image of neurite outgrowth in Ad-GFP-2A-iCre-infected cells. Neurons are labelled with beta III tubulin and viral transfection indicated by a GFP-Cre-expressing viral construct. Long arrows indicate Cre recombinase-expressing cells and short arrows indicate Cre recombinase non-expressing cells. Note the lesser neurite outgrowth in cells without GFP-Cre (e). Low-power image of neurite outgrowth in Ad-GFP (control)-infected cells. Outgrowth was less extensive in this neuronal population (f) (Bar=500 μm fore,f). High-power image of neurite outgrowth in Ad-GFP-2A-iCre-infected cells. Long arrows indicate Cre recombinase expressed cells and short arrows indicate Cre recombinase non-expressed cells (g) (Bar=100 μm forg,h). Higher-power image of neurite outgrowth in Ad-(control)-infected cells (h). Figure 4: Conditional knockdown of Rb1 in adult sensory neurons from Rb1-floxed mice is associated with enhanced neurite outgrowth. Conditional knockdown of Rb1 is associated with rises in neurite outgrowth, maximum process length, numbers of processes (neurites) and numbers of branches ( a – d ) (*** P <0.001 for a , ** P =0.001 for b , ** P <0.01 for c , * P <0.05 for d ; n =6/group; unpaired two-tailed Student’s t -tests). Values are means±s.e.m. Low-power image of neurite outgrowth in Ad-GFP-2A-iCre-infected cells. Neurons are labelled with beta III tubulin and viral transfection indicated by a GFP-Cre-expressing viral construct. Long arrows indicate Cre recombinase-expressing cells and short arrows indicate Cre recombinase non-expressing cells. Note the lesser neurite outgrowth in cells without GFP-Cre ( e ). Low-power image of neurite outgrowth in Ad-GFP (control)-infected cells. Outgrowth was less extensive in this neuronal population ( f ) (Bar=500 μm for e , f ). High-power image of neurite outgrowth in Ad-GFP-2A-iCre-infected cells. Long arrows indicate Cre recombinase expressed cells and short arrows indicate Cre recombinase non-expressed cells ( g ) (Bar=100 μm for g , h ). Higher-power image of neurite outgrowth in Ad-(control)-infected cells ( h ). Full size image Since Rb knockdown has been linked to evidence of apoptosis in some published models [11] , we analysed the levels, in neurons exposed to Rb knockdown or deletion, of phosphohistone H2A.X and activated caspase 3, putative markers of DNA double-stranded break and apoptosis, respectively ( Fig. 5a–c ; Supplementary Fig. 4 ). We found no difference in the levels of phosphohistone H2A.X in the control and Rb siRNA-treated cells. Whereas baseline levels of phosphohistone H2A.X and activated caspase 3 were slightly higher, qualitatively, in adenovirus-exposed neurons, levels were similar in neurons treated with Cre recombinase compared with controls. Moreover, the presence of these molecular markers did not correlate with any morphological evidence of impaired viability; processes were intact and had adequate branching capability. Expression of activated caspase 3 has been previously described in intact and viable DRG neurons [14] . As a quantitative measure of cell death, we used an lactate dehyrogenase (LDH) release toxicity assay and compared Rb-floxed neurons from mice transfected with Cre to control transfections and also compared rat neurons exposed with Rb1 siRNA to those exposed to scrambled sequence control siRNA. Neither Rb1 knockdown strategy was associated with LDH release that exceeded controls, indicating an absence of significant cell death ( Fig. 5d ). Taken together, these results did not identify evidence of cell death associated with Rb knockdown in the time frames and conditions examined here. Selective loss of neurons did not account for the readouts identifying substantial rises in neurite outgrowth identified in our system. 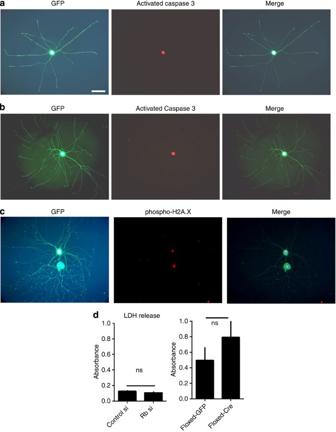Figure 5: Transient knockdown of Rb in sensory neurons is not associated with increased cell death. While activated caspase 3 expression was observed in neurons in both control (Ad-GFP) (a) and Cre-expressing (Ad-GFP-2A-iCre) (b) treated cells, neurons had normal morphology and intact neurite outgrowth. Expression of activated caspase 3 has been previously reported in significant numbers of intact and viable neurons14. Expression of phospho-H2A.X in Ad-GFP-2A-iCre-treated cells (c) was also associated with intact and viable neuron morphology (and seeSupplementary Fig. 4) (Bar=100 μma–c). LDH release (d) was similar (ns;n=4, rats; unpaired two-tailed Student’st-test) in adult rat DRG neurons exposed to scrambled siRNA compared with Rb siRNA (as inFig. 3) and in adult mouse Rb-floxed neurons (ns;n=3; unpaired two-tailed Student’st-test) exposed to control adenovirus compared to adenovirus expressing Cre recombinase. Values are means±s.e.m. Figure 5: Transient knockdown of Rb in sensory neurons is not associated with increased cell death. While activated caspase 3 expression was observed in neurons in both control (Ad-GFP) ( a ) and Cre-expressing (Ad-GFP-2A-iCre) ( b ) treated cells, neurons had normal morphology and intact neurite outgrowth. Expression of activated caspase 3 has been previously reported in significant numbers of intact and viable neurons [14] . Expression of phospho-H2A.X in Ad-GFP-2A-iCre-treated cells ( c ) was also associated with intact and viable neuron morphology (and see Supplementary Fig. 4 ) (Bar=100 μm a – c ). LDH release ( d ) was similar (ns; n =4, rats; unpaired two-tailed Student’s t- test) in adult rat DRG neurons exposed to scrambled siRNA compared with Rb siRNA (as in Fig. 3 ) and in adult mouse Rb-floxed neurons (ns; n =3; unpaired two-tailed Student’s t- test) exposed to control adenovirus compared to adenovirus expressing Cre recombinase. Values are means±s.e.m. Full size image Rb knockdown-related targets We next examined several candidate plasticity proteins that are known targets of Rb. Neurons undergoing Rb knockdown were harvested and protein lysates were examined. Pak1, CDK5 and PPARυ have previously been reported to be downstream effectors of Rb in multiple systems and, interestingly, these molecules were shown to have possible roles on nerve regeneration [15] , [16] , [17] , [18] , [19] , [20] . Particular consideration was given to the PI3K-Akt pathway, well known to enhance outgrowth in response to insulin, other growth factors and PTEN inhibition [9] , [21] ( Fig. 6 ; Supplementary Fig. 5a,b ). Changes in the levels of pAkt however, the key effector of this pathway, were not identified. Pak1 is a second messenger for Rac1, a GTPase associated with increased growth cone extension. Its levels were not altered by Rb knockdown. Finally, we did not detect a significant change, beyond a mild trend towards downregulation, in CDK5, a neuronal specific cyclin-dependent kinase. CDK5/p35 may operate upstream of Rb [22] . In contrast to these results, we identified an unexpected but consistent upregulation of PPARυ protein and mRNA in sensory neurons following knockdown of Rb ( Fig. 6b–i ). This change was verified through two differing siRNA constructs. We next confirmed using immunocytochemistry that PPARυ was expressed in adult sensory neurons, located in their cytoplasm, nucleus and to a lesser extent in their neurite processes ( Fig. 6i ). After axotomy injury, there was a nonsignificant trend towards its upregulation ( Supplementary Figs 1 and 2 ). Overall, the findings identified a new neuronal target, PPARυ, in adult neurons having undergone Rb knockdown. 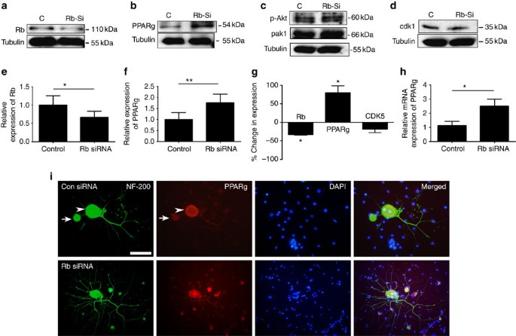Figure 6: Knockdown of Rb1 increases the expression of PPARυ. Rb1 siRNA is associated with knockdown of the Rb1 protein in dissociated adult sensory neurons (a) and a rise in PPARυ expression (b) without changes in pAkt, Pak1 or CDK5 (c,d). Quantitation of western blot data showing declines in Rb (e) (*P<0.05;n=4; paired two-tailed Student’st-test) and rises in PPARυ(f) (**P<0.01;n=4; paired two-tailed Student’st-test) and relative changes in expression (g). Rb siRNA was also associated with a rise in PPARυ mRNA (h) (*P=0.048;n=four control/scrambled, three Rb siRNA; unpaired Mann–Whitney two-tailed test). Values are means±s.e.m. Images (i) of dissociated adult sensory neurons exposed to scrambled (Con, top panels) or Rb siRNA and labelled with antibodies to neurofilament (green,NF200), PPARυ (red) and colabelled with a nuclear stain (blue, DAPI). Note the greater neurite outgrowth of neurons exposed to Rb siRNA and the qualitative increase in PPARυ-staining intensity. Bar=100 μm. Figure 6: Knockdown of Rb1 increases the expression of PPARυ. Rb1 siRNA is associated with knockdown of the Rb1 protein in dissociated adult sensory neurons ( a ) and a rise in PPARυ expression ( b ) without changes in pAkt, Pak1 or CDK5 ( c , d ). Quantitation of western blot data showing declines in Rb ( e ) (* P <0.05; n =4; paired two-tailed Student’s t -test) and rises in PPARυ( f ) (** P <0.01; n =4; paired two-tailed Student’s t- test) and relative changes in expression ( g ). Rb siRNA was also associated with a rise in PPARυ mRNA ( h ) (* P =0.048; n =four control/scrambled, three Rb siRNA; unpaired Mann–Whitney two-tailed test). Values are means±s.e.m. Images ( i ) of dissociated adult sensory neurons exposed to scrambled (Con, top panels) or Rb siRNA and labelled with antibodies to neurofilament (green,NF200), PPARυ (red) and colabelled with a nuclear stain (blue, DAPI). Note the greater neurite outgrowth of neurons exposed to Rb siRNA and the qualitative increase in PPARυ-staining intensity. Bar=100 μm. Full size image PPARυ contributes to Rb knockdown plasticity To test the potential significance of PPARυ upregulation, we examined neurite outgrowth and branching in neurons with combined Rb knockdown and PPARυ antagonism. GW9662, a selective competitive pharmacological antagonist of PPARυ dose-dependently inhibited the enhancement of neurite outgrowth associated with Rb siRNA ( Fig. 7a–e ; Supplementary Fig. 6 ). Outgrowth inhibition included total neurite outgrowth, numbers of primary neurites, the longest neurite measured and the number of neurite branches. At its higher dose, GW9662 suppressed outgrowth values below those of controls, suggesting that its constitutive actions might be important for baseline neuron growth. In contrast to the suppression of growth by the PPARυ antagonist, a PPARυ agonist, 15PGJ2, at 100 nM, increased overall outgrowth and the length of the longest neurites ( Fig. 7f ). The impact of the agonist, however, was less robust than that of Rb knockdown and did not include an impact on neurite branching. Only nonsignificant trends towards increased branch numbers were observed ( Fig. 7f ). Taken together, the findings provided evidence that PPARυ acts downstream of Rb and may contribute towards plasticity when its repression by Rb is relieved. 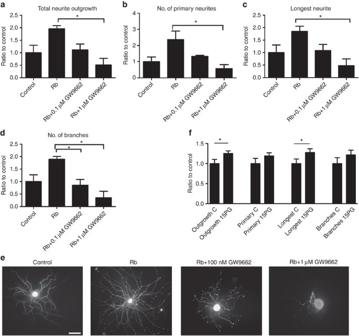Figure 7: Neurite plasticity following Rb1 knockdown is blocked by a PPARυ antagonist. Dissociated uninjured (non-preconditioned) adult sensory neurons exposed to one of two differing Rb1 siRNA constructs showed enhanced growth. Bars indicate control neurite outgrowth, Rb1 siRNA outgrowth and Rb1 siRNA outgrowth with GW9662 at 0.1 or 1.0 μM. Rb1 siRNA is associated with rises in total neurite outgrowth (a) (*P<0.05;n=3; analysis of varianceP<0.05;post hocTukey), greater numbers of primary neurites (b) (*P<0.05;n=3; ANOVAP<0.05;post hocTukey), longer neurites (c) (*P<0.05;n=3; ANOVAP<0.05;post hoc Tukey) and rises in the number of neurite branches (d) (*P<0.05;n=3; ANOVAP<0.01;post hocTukey). The panel below (e) illustrates examples of sensory neurons exposed to an Rb1 siRNA constructs without or with two differing doses of GW9662 (Bar=10 μm, Bar=100 μm). In contrast, exposure of dissociated adult sensory neurons to a PPARυ agonist (f), 15PGJ2 at 100 nM was associated with rises in total neurite outgrowth (*P<0.01;n=7; paired two-tailed Student’st-test) and in the length of the longest neurite (*P<0.05;n=7; paired two-tailed Student’st-test). Values are means±s.e.m. Figure 7: Neurite plasticity following Rb1 knockdown is blocked by a PPARυ antagonist. Dissociated uninjured (non-preconditioned) adult sensory neurons exposed to one of two differing Rb1 siRNA constructs showed enhanced growth. Bars indicate control neurite outgrowth, Rb1 siRNA outgrowth and Rb1 siRNA outgrowth with GW9662 at 0.1 or 1.0 μM. Rb1 siRNA is associated with rises in total neurite outgrowth ( a ) (* P <0.05; n =3; analysis of variance P <0.05; post hoc Tukey), greater numbers of primary neurites ( b ) (* P <0.05; n =3; ANOVA P <0.05; post hoc Tukey), longer neurites ( c ) (* P <0.05; n =3; ANOVA P <0.05; post ho c Tukey) and rises in the number of neurite branches ( d ) (* P <0.05; n =3; ANOVA P <0.01; post hoc Tukey). The panel below ( e ) illustrates examples of sensory neurons exposed to an Rb1 siRNA constructs without or with two differing doses of GW9662 (Bar=10 μm, Bar=100 μm). In contrast, exposure of dissociated adult sensory neurons to a PPARυ agonist ( f ), 15PGJ2 at 100 nM was associated with rises in total neurite outgrowth (* P <0.01; n =7; paired two-tailed Student’s t -test) and in the length of the longest neurite (* P <0.05; n =7; paired two-tailed Student’s t- test). Values are means±s.e.m. Full size image Rb knockdown improves outgrowth after axotomy To test whether Rb knockdown might be associated with altered behaviour of regenerating axons in vivo , we examined their outgrowth properties following exposure to local administration of siRNA delivered to injured nerve trunks. In previous studies we have shown that local nonviral delivery of siRNAs provides specific and potent actions both at the site of application but also through retrograde uptake by neurons, when applied to outgrowing axons and their accompanying SCs [7] , [23] , [24] . Despite assumptions otherwise, transected peripheral neurons are highly hesitant in their outgrowth properties and limited to slow and staggered advancements beyond the injured zone [1] . Only 10% of axons are estimated to successfully cross these types of injury zones, even with microfascicular repair [5] . An improvement in this success rate could translate into improved regenerative outcomes. After transection of the sciatic nerves in adult rats, a gap of 3–5 mm is formed from retraction of the distal and proximal stumps, similar to clinical scenarios in human nerve injuries. In our experimental paradigm, a silicone conduit was inserted within the retraction gap and connected to the proximal and distal stumps, as used in clinical nerve repair. A side arm of the conduit was connected to a subcutaneous access port to allow repeated installation of local siRNAs into the regenerative microenvironment, and analysis was carried out of the extent of axon outgrowth from the proximal stump ( Fig. 8a,b ). Both the approach and the impact of this strategy have been extensively validated in previous work [25] , [26] . After transection and conduit placement, injections of 0.2 ml were given on days 0, 1, 3 and 5 for Rb or scrambled siRNA (2 μg per injection). Bridges were processed for immunohistochemistry and probed for the axon marker NF200 (1:800) and a marker for accompanying activated SCs, glial fibrillary acidic protein (GFAP; 1:250). At the beginning of the outgrowth zone in the first separate high-power field (400 μm), a clear demarcation could be recognized in the overall structure of the nerve trunk, and the onset of regenerative neurofilament containing axon profiles. Starting at the distal edge of the proximal stump, we counted profiles in a line perpendicular to the direction of the bridge in serial fields distally in high-power fields every 270 μm until reaching the last field expressing the heavy-chain neurofilament protein, NF200 (neurofilament; Fig. 8b–d ). 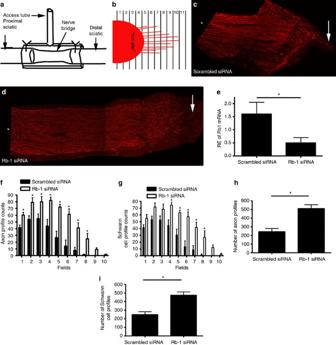Figure 8: Knockdown of Rb1 increases axon regenerationin vivo. Regeneration conduit showing where the proximal and distal sciatic nerves are sutured into the chamber (a). To the right is a schematic of the field quantification used for regenerating axon length (b). Longitudinal section of the sciatic nerve labelled with NF200, 7 days after treatment with scrambled siRNA in the regeneration chamber (c). Longitudinal section of sciatic nerve 7 days after treatment with Rb1 siRNA (asterisk denotes the side of the proximal stump, arrow points to the longest regenerating axon(d)) (forc,dBar=200 μm). qRT–PCR showed a decrease in Rb1 mRNA with Alexa-488 Rb1 siRNA in the chamber (*P<0.05,n=5; unpaired one-tailed Student’st-test) (e). Axon profile count in fields from the injury site (*P<0.05,n=4; unpaired two-tailed Student’st-test) (f). Total axon counts for regenerating tip for scrambled and Rb1 siRNA (*P<0.005,n=4; unpaired two-tailed Student’st-test) (h). Schwann cell profile counts from the injury site (*P<0.05,n=4; unpaired two-tailed Student’st-test) (g). Total Schwann cell counts for regenerating tip for scrambled and Rb1 siRNA (P<0.005,n=4; unpaired two-tailed Student’st-test) (i). Values are means±s.e.m. Figure 8: Knockdown of Rb1 increases axon regeneration in vivo . Regeneration conduit showing where the proximal and distal sciatic nerves are sutured into the chamber ( a ). To the right is a schematic of the field quantification used for regenerating axon length ( b ). Longitudinal section of the sciatic nerve labelled with NF200, 7 days after treatment with scrambled siRNA in the regeneration chamber ( c ). Longitudinal section of sciatic nerve 7 days after treatment with Rb1 siRNA (asterisk denotes the side of the proximal stump, arrow points to the longest regenerating axon( d )) (for c , d Bar=200 μm). qRT–PCR showed a decrease in Rb1 mRNA with Alexa-488 Rb1 siRNA in the chamber (* P <0.05, n =5; unpaired one-tailed Student’s t -test) ( e ). Axon profile count in fields from the injury site (* P <0.05, n =4; unpaired two-tailed Student’s t -test) ( f ). Total axon counts for regenerating tip for scrambled and Rb1 siRNA (* P <0.005, n =4; unpaired two-tailed Student’s t -test) ( h ). Schwann cell profile counts from the injury site (* P <0.05, n =4; unpaired two-tailed Student’s t -test) ( g ). Total Schwann cell counts for regenerating tip for scrambled and Rb1 siRNA ( P <0.005, n =4; unpaired two-tailed Student’s t- test) ( i ). Values are means±s.e.m. Full size image As with the in vitro experiments, local in vivo siRNA was associated with knockdown of Rb1 siRNA within the axon outgrowth injury zone ( Fig. 8e ). In response to knockdown we observed a substantial rise in the numbers of outgrowing axons in most fields distal to the transection zone as well as a greater outgrowth distally ( Fig. 8c,d,f,h ). The outgrowth in proximal fields indicated a vigorous sprouting response while individual axons also extended greater distances into the conduit. A separate analysis of SC outgrowth similarly confirmed substantially larger numbers of profiles in both proximal and distal fields beyond the transection zone ( Fig. 8g,i ). Overall, these findings extended the observations in vitro that Rb knockdown can be translated into a meaningful and robust in vivo paradigm, with a substantial impact on outgrowth. The findings also confirm our previous conclusions that closely knit axon–SC partnerships allow strategies that ostensibly only support one or other of these partners to ultimately influence growth in both of them [24] , [25] . Rb knockdown improves recovery from nerve injury We next asked whether in vitro axon sprouting and early in vivo outgrowth, as demonstrated above, translate into longer-term recovery from nerve injury. We examined behavioural indices of sensory and motor axon regrowth in mice following a sciatic nerve crush injury with or without Rb knockdown using local administration of siRNA. Mice were chosen for these experiments because their shorter nerve trajectories allow more rapid evaluation of recovery of function. We also aimed to determine whether the putative impact of Rb knockdown could be demonstrated in a second, separate animal model. siRNA (Rb1 or scrambled) solution was applied to the crush area immediately after crush then serially for 5 days both at the crush site and into the distal territory of the nerve in the hindpaw. We confirmed that this approach, also described in previous work, knocked down the Rb mRNA transcript both locally within the injured nerve and in the ipsilateral DRG (there was a nonsignificant trend towards increased PPARυ mRNA in the DRG ( Supplementary Fig. 4 )). As demonstrated using other siRNA constructs without viral delivery, DRG knockdown occurs from retrograde transport of the siRNA [24] . Measures of hindpaw grip strength, mechanical sensitivity and thermal sensitivity were carried out at baseline and then repeated at 14 and 28 days. By 14 days mice exposed to scrambled siRNA had lower hindpaw grip strength than pre-injury and also had mechanical hypoalgesia and thermal hyperalgesia, all expected features of early but partial recovery to nerve injury ( Fig. 9 ). In contrast, mice exposed to local Rb siRNA had a more rapid recovery of hindpaw grip strength, earlier resolution of mechanical hypoalgesia and prevention of thermal hyperalgesia. Regenerating axons exposed to Rb siRNA also had more rapid recovery of sensory but not motor conduction velocity. Taken together, these results provide evidence that Rb knockdown is associated with functional indices of regeneration following nerve injury. They support our working hypothesis that in vitro and early in vivo outgrowth indices of axon growth predict functional benefits of regenerative strategies. 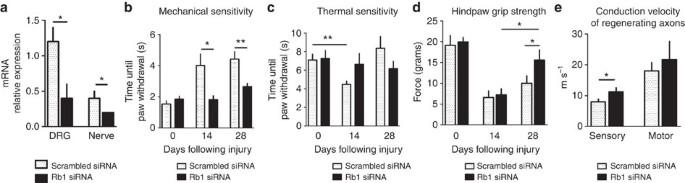Figure 9: Local knockdown of Rb1 improves the functional recovery following nerve injury. Outbred mice underwent a crush injury of the sciatic nerve under anaesthesia. Immediately after the injury, and for 5 additional days, the injury site was administered either scrambled sequence siRNA or siRNA directed to Rb1. Rb1 knockdown was confirmed both at the level of the ipsilateral DRG housing the perikarya of the sciatic nerve sensory branches and locally at the injury site 7 days after injury (a) (*P<0.05 for DRG;n=7 scrambled/DRG, four Rb siRNA/DRG; unpaired two-tailed Student’st-test; *P<0.05 for nerve;n=8 scrambled/nerve, 4/Rb1 siRNA/nerve; unpaired two-tailed Student’st-test with Welch’s correction). Serial studies of mechanical sensitivity of the ipsilateral hindpaw indicated a rapid improvement in sensitivity in the Rb1 siRNA group at both 14 and 28 days following injury (b) (*P<0.05 at 14 days and **P<0.005 at 28 days;n=8–10; unpaired two-tailed Student’st-test). Thermal sensitivity studies identified injury-related hyperalgesia in the scrambled siRNA group at 14 days, but not the Rb1 siRNA group. By 28 days, both groups had recovered, but there was a nonsignificant trend towards more sensitivity in the Rb1 siRNA-treated group (c) (*P<0.005;n=8–10; unpaired two-tailed Student’st-test). After injury there was an expected decline in hindpaw grip power at 14 days. By 28 days, greater recovery in hindpaw power was identified in mice treated with Rb siRNA (d) (*P<0.05 14 versus 28 days for Rb1 siRNA;n=8=10; unpaired two-tailed Student’st-test; *P<0.05 for 28 days;n=8–10; unpaired one-tailed Student’st-test). Multifibre sciatic–tibial motor conduction studies identified better recovery in sensory conduction velocity at 28 days post injury. No impact on motor conduction velocity was identified (e) (*P<0.05 for sensory conduction velocity;n=8–9; unpaired one-tailed Student’st-test). Values are means±s.e.m. Figure 9: Local knockdown of Rb1 improves the functional recovery following nerve injury. Outbred mice underwent a crush injury of the sciatic nerve under anaesthesia. Immediately after the injury, and for 5 additional days, the injury site was administered either scrambled sequence siRNA or siRNA directed to Rb1. Rb1 knockdown was confirmed both at the level of the ipsilateral DRG housing the perikarya of the sciatic nerve sensory branches and locally at the injury site 7 days after injury ( a ) (* P <0.05 for DRG; n =7 scrambled/DRG, four Rb siRNA/DRG; unpaired two-tailed Student’s t -test; * P <0.05 for nerve; n =8 scrambled/nerve, 4/Rb1 siRNA/nerve; unpaired two-tailed Student’s t- test with Welch’s correction). Serial studies of mechanical sensitivity of the ipsilateral hindpaw indicated a rapid improvement in sensitivity in the Rb1 siRNA group at both 14 and 28 days following injury ( b ) (* P <0.05 at 14 days and ** P <0.005 at 28 days; n =8–10; unpaired two-tailed Student’s t- test). Thermal sensitivity studies identified injury-related hyperalgesia in the scrambled siRNA group at 14 days, but not the Rb1 siRNA group. By 28 days, both groups had recovered, but there was a nonsignificant trend towards more sensitivity in the Rb1 siRNA-treated group ( c ) (* P <0.005; n =8–10; unpaired two-tailed Student’s t -test). After injury there was an expected decline in hindpaw grip power at 14 days. By 28 days, greater recovery in hindpaw power was identified in mice treated with Rb siRNA ( d ) (* P <0.05 14 versus 28 days for Rb1 siRNA; n =8=10; unpaired two-tailed Student’s t -test; * P <0.05 for 28 days; n =8–10; unpaired one-tailed Student’s t -test). Multifibre sciatic–tibial motor conduction studies identified better recovery in sensory conduction velocity at 28 days post injury. No impact on motor conduction velocity was identified ( e ) (* P <0.05 for sensory conduction velocity; n =8–9; unpaired one-tailed Student’s t -test). Values are means±s.e.m. Full size image An overriding conclusion from our work is its support for the concept that manipulation of tumour suppressor pathways offers unexplored potential to manipulate growth patterns in adult neurons. In this context, Rb is a very well-known representative; however, its expression and role in adult neurons and their growth have not been previously explored. Our findings parallel how peripheral neurons respond to suppression of another tumour suppressor molecule, PTEN [7] . Both knockdown of Rb in this work and PTEN previously were associated with robust neurite outgrowth in vivo , particularly prominent in preconditioned neurons. ‘Preconditioning’ refers to the property of neurons to ramp up their regenerative activity in response to a prior lesion and is associated with substantial rises in outgrowth. Exploitation of preconditioned pathways has been a goal of regenerative investigators for some years, in part mimicked by rises in neuronal cAMP levels [27] . Remarkably, both PTEN and Rb suppression had impacts that were additive to preconditioning, an exciting form of plasticity that, if exploited, may have wide applicability. Both approaches also translated their impacts into benefits on outgrowth from transected peripheral nerve trunks. We believe that the responses we identified to Rb knockdown or silencing were neuronal and were not mediated by an impact on glial cells. This was supported by the direct findings involving neurons in vitro , and Rb’s very limited expression in glial cells. The retrograde knockdown of Rb we observed in DRGs after crush injury and local delivery of Rb siRNA suggests retrograde axonal transport of the siRNA in neurons. Unlike PTEN knockdown, the mechanism of Rb knockdown-mediated plasticity does not appear to involve upregulated pAkt. While this finding excludes a well-known neuron plasticity pathway, Sears and Nevins [10] suggest that pAkt may instead operate upstream of Rb. If that is the case, knockdown of Rb may have derepressed a constitutive action of pAkt on growth. Its robust actions however suggest a more active mechanism. Similarly, by acting upstream of Rb, MEK-ERK-Myc are less likely to be implicated in how Rb knockdown enhances plasticity. To search for other known targets of Rb that might instead mediate its actions, we identified upregulation of PPARυ in neurons. PPARυ antagonism blocked the plasticity associated with Rb knockdown and a PPARυ agonist increased neurite outgrowth. The involvement of PPARυ, however, does not exclude the possibility that it acts parallel to other unexplored pathways involved in growth cone advancement. This is possible since the PPARυ agonist alone had a less robust impact on both outgrowth but particularly on branching than Rb knockdown alone. Changes in PPARυ levels in response to Rb manipulation are described in other systems [17] , [28] , [29] . For example, PPARυ may render CNS neuroprotection [30] , [31] and is expressed in injured sciatic nerves. The latter form of expression has been linked to growth on inhibitor myelin substrates [20] , [32] . Despite these findings, its role in adult nerve regeneration has not been otherwise examined. Rb inhibits E2F transcriptional activity where E2F1 and E2F3 appear to promote PPARυ transcription, whereas E2F4 represses it [33] , [34] . Thus under our experimental conditions, Rb silencing-mediated activation of E2F isoforms might have enhanced the expression of PPARυ. Over threshold activation of E2F can direct cells to other fates also, leading to death of mature neurons by stimulating cell cycle entry [22] . Thus, the silencing of the Rb protein (~50%) achieved under our experimental conditions may represent optimal activation of E2F, prompting mature neurons to facilitate axon regeneration. While the acceleration of outgrowth of both axons and SCs beyond their severed nerve trunks is a critical first step towards improving the outcome of these lesions, our data also suggest that this outgrowth enhances functional and longer-term regenerative outcomes. The potential role of Rb knockdown in central axon pathways has not yet been explored, sites with yet greater regenerative restraints. Despite this caveat, we believe that both Rb and PPARυ are important and novel targets for newer regenerative strategies. In addition to identifying two new molecular players in neuronal regeneration, our findings indicate the strong possibility that a wider range of novel shared oncogenic and neuronal proteins and pathways exist. Their manipulation in a localized and temporary context may offer opportunities to improve neurological outcome. Animals and preconditioning lesion experiments Adult male Sprague–Dawley rats (Charles River Laboratory, Senneville, Canada) with an initial weight of 200–300 g were used and all animal studies were approved by the University of Calgary Animal Care Committee. For preconditioning, the sciatic nerve was cut at the mid-thigh level under aseptic conditions. A sham injury in separate animals was performed by exposing but not severing the sciatic nerve. Rb-floxed mice breeder pairs (FVB; 129- Rb1 tm2Brn ) were obtained from the National Cancer Institute mouse repository. The mice were propagated in the in-house animal care facility in the University of Calgary. For in vivo regeneration experiments and additional in vitro sensory neuron assays, we used male CD1 mice (Charles River Laboratory) with an initial weight of 17–21 g . Quantitative reverse transcription-polymerase chain reaction Total RNA was extracted from tissues using Trizol reagent and PCR primers that were designed using software Primer Express 2.0 (Applied Biosystems, Foster City, CA, USA): Cyclophilin F 5′-TGTGCCAGGGTGGTGACTT-3′ R 5′-TCAAATTTCTCTCCGTAGATGGACTT-3′ RPLP0 F 5′-TACCTGCTCAGAACACCGGTCT-3′ R 5′-GCACATCGCTCAGGATTTCAA-3′ Rb1 F 5′-TTACAGTATGCCTCCACCAGGC-3′ R 5′-TTACCTCCAGGAATCCGCAAG-3′ PPARg (rat) F5′-TTCAAACTCCCTCATGGCCA-3′ R 5′-GTTCTTCGGAAAAAACCCTTGC-3′ PPARg (mouse) F5′-GATCATCTACACGATGCTGGCC-3′ R 5′-TTCCGCAGGCTTTTGAGGA-3′ Cyclophilin, RPLP0 or Rb1 products were labelled with SybrGreen (Invitrogen, Burlington, Ontario, Canada). All reactions were performed in duplicate using an ABI PRISM 7000 Sequence Detection System (Applied Biosystems) and analysed using the 2 ΔΔ Cycle Threshold method. Results were presented as the fold induction of mRNA in L4-L5 DRG neurons or sciatic nerve normalized to Cyclophilin or RPLP0, and compared to normal, uninjured L4-L5 DRG neurons or sciatic nerve (defined as 1.0-fold). Western immunoblot Ten micrograms of total protein, extracted from adult sensory neuronal cultures treated with scrambled siRNA or Rb siRNA, were loaded for SDS–PAGE. Membrane was incubated overnight with the respective antibodies: Rb, 1:500 in 2% bovine serum albumin (BSA) in TBST (2% TBST), rabbit polyclonal, Santa Cruz; PPARυ, 1:400 in 2% TBST, mouse monoclonal, Santa Cruz; pAkt, 1:500 in 2% TBST, rabbit monoclonal, Cell Signalling; pak1, 1:1,000 in 2% TBST, rabbit monoclonal, Abcam; cdk5; 1:500 in 2% TBST; rabbit polyclonal; Santa Cruz. Tubulin (1:3,000 in 2% TBST; mouse monoclonal, Sigma) and actin (1:1,000 in 2% TBST; mouse monoclonal, Millipore) were used as the loading controls. Quantification of bands was through Adobe Photoshop and the band densities were normalized with those of the loading control. Antibodies and immunohistochemistry Harvested L4, L5 DRGs and sciatic nerve (normal or proximal and distal to transection) were probed for Rb (1:200, Santa Cruz Biotechnology, sc-50), and double-labelled with S100β (1:200, Sigma), or with NF200 (1:400, Rabbit polyclonal, Sigma-Aldrich) for 48 h, and then rinsed three times in phosphate-buffered saline. Secondary antibodies were sheep antimouse IgG CY3 conjugate (1:100, Sigma) and Alexa Fluor 488 goat anti-rabbit IgG (H+L) conjugate (1:500, Cedarlane, Horby, Canada). Dissociated DRG cultures were labelled with Rb (1:200), PPARυ (1:50, Mouse monoclonal, Cell Signalling), NF200 (1:500), activated caspase 3 (1:200); phospho-H2A.X (1:200); and β tubulin III (1:100). Antibodies to activated caspase 3 and phosphohistone H2A.X (Ser 139) were purchased from Trevigen and Millipore, respectively. β tubulin III antibody was purchased from Sigma. Adult sensory neuron cultures Dissociated adult sensory neuron culture protocols using rat DRG were as described previously [7] . Briefly, rats were anaesthetised with Isoflurane (Abbot Laboratories) and then killed 3 days following the conditioning lesion or sham surgery. L4-L5 DRGs were removed from the rats and placed into L15 (Invitrogen) medium (one rat (two DRGs) per condition per culture day were plated on a four-chamber slide). The DRGs were rinsed and then transferred to a tube containing 2 ml 0.1% collagenase (Invitrogen)/L15. Following incubation at 37 °C, the DRGs were placed into single-cell suspension by triturating. The single-cell suspension was spun and washed three times in 2 ml L15. After the final spin, the cells were resuspended in L15 and passed through a 70-μm mesh (VWR International Co.) and then placed in 500 μl L15 enriched with 1:100 dilution of N2 supplement (Invitrogen) and 0.1% BSA (Sigma) and placed into a culture medium of Dulbecco’s Modified Eagle Medium/F12 (DMEM/F12; Invitrogen) +1:100 dilution N2, 0.5–0.8% BSA and 0.2 ng ml −1 NGF (Cedarlane Laboratories) plus 50U Penicillin × ml −1 , 50U Streptomycin × ml −1 (Invitrogen) and plated on poly-L-lysine (Sigma-Aldrich) and 10 μg ml −1 mouse laminin (Invitrogen)-coated plates. In separate experiments, Alexa-488-tagged Rb or scrambled siRNA (Qiagen, Valencia, CA, USA) were added to the medium at 20 nM along with the HiPerFect transfection reagent according to the HiPerFect handbook (Qiagen). Cells were grown for 18–20 h and analysed for neurite extension (mean per neuron), number of primary neurites (defined as processes extending from the soma), length of the longest neurite, number of branches (defined as a branch point in a primary neurite) and cell body area quantified by the MetaXpress software and an observer blinded to their condition (Molecular Devices, Sunnyvale, CA, USA). Between 40 and 60 neurons were analysed per condition and per culture day (four culture days, 240 neurons total for each condition). Three–four rats/condition were routinely used. For siRNA experiments, neurons were quantified if they contained the Alexa 488 fluorescent siRNA tag. For PPARυ antagonist studies, the PPARυ-specific antagonist GW9662 (Sigma), at 0.1 and 1 μM, was added to the culture with the Rb siRNA; neurite outgrowth studies were performed at 36 h. For PPARυ agonist studies, the specific PPARυ agonist, 15PGJ2, at 100 nM, was added to the culture while plating the cells; neurite outgrowth studies were performed at 36 h. The following Rb1 siRNA target sequences were used (Qiagen) for the in vitro work: 5′-TAGCATATCTCCGACTAAATA-3′ (rat studies, sequence 1) 5′-AAGGAGCACGAGTGTAATGTA-3′ (rat studies, sequence 2) 5′-ATCGAGGTTCTCTGTAAAGAA-3′ (mouse studies). For E2F1, the siRNA target sequence (Qiagen) used was: 5′-ACAAATGGTCATAGTGATCAA-3′. Adenovirus particles expressing GFP or Cre recombinase or both were purchased from Vector Biolabs. Cisplatin was purchased from Sigma. Adult mice (FVB; 129- Rb1 tm2Brn ; 6-weeks old) were anaesthetized using isoflurane and were killed by cardiac puncture. DRGs at the lumbar and thoracic regions were harvested from both sides of the spinal column. The isolated DRGs were placed in 0.1% collagenase and incubated at 37 °C for 45 min. The individual cells were then dissociated by repeated pipetting of the DRGs in collagenase solution followed by centrifugation (800 r.p.m. ; 6 min) to pellet down the cells. The cell suspension was then laid over 15% BSA and centrifuged to remove the debris formed as a middle layer. The cell pellet was suspended in culture media containing recommended growth factors and 50 U ml −1 penicillin and streptomycin. The cells were infected with either Ad-GFP or Ad-CMV-Cre particles (500 p.f.u. per cell) at the time of seeding in four-well chamber slides or coverslips precoated with poly-l-lysine and laminin. The cells were harvested at 24 h post infection and total mRNA was isolated. For neurite outgrowth studies and other immunocytochemical analyses, the cells were fixed at 48 h post infection. In separate experiments, the cells were infected with Ad-GFP-2A-iCre particles that express both Cre recombinase and GFP. Cisplatin was dissolved in saline and the primary sensory neuronal cells were incubated with 20 μg ml −1 cisplatin for 24 h. LDH toxicity assay LDH release from sensory neurons in vitro was utilized as a measure of cell death (Sigma) according to the manufacturer’s instructions. Briefly, the cell-culture supernatant and the LDH assay mixture were mixed in 1:2 ratios and incubated for 30 min at room temperature. The reaction was terminated using 1 N HCl and the absorbance was read at 490 nm. Absorbance at 690 nm was also read and used for the background correction. Regeneration experiments Our experimental design for analysing early outgrowth of axons from transected rat sciatic nerve has been previously described [7] , [26] . A 3-cm incision was made along the length of the lateral aspect of the left thigh, beginning at the sciatic notch and ending near the knee. A second incision was made on the dorsal aspect of the animal superior to the scapulae and parallel to the vertebral column to facilitate insertion of a microinjection port (MIP). Next, blunt forceps were used to tunnel through the subdermal fascia between posterior and anterior incisions. The jaws of the forceps were then used to pull the catheter of the MIP from its implantation site to the incision at the hindlimb. The catheter of the MIP was glued into the access tube of the T-chamber using cyanoacrylate cement. Blunt dissection was performed to expose and mobilize the left sciatic nerve, which was transected at the mid-thigh level using an 11-0 scalpel blade. The proximal and distal stumps of the nerve were then secured into the ends of the nerve chamber using a single 9-0 nylon (Ethicon) suture through the epineurium of each stump, leaving a gap (3 mm) between stumps. Before closing the wound, a single 4-0 silk suture (Ethicon) was applied to secure the T-intersection of the tube to underlying muscle and a second suture was used to reattach the retracted gluteal muscle. Finally, a continuous suture (4-0 silk) was used to close both incisions. At end point, nerve chambers were harvested by transection of proximal and distal nerve segments several millimetres from the nerve chamber. Removal of the epineurial sutures freed the regenerate, and the nerve bridge (regenerate) was obtained by lightly pulling the nerve through the chamber. Injections of 0.2 ml were given on days 0, 1, 3 and 5 for Rb and scrambled siRNA (2 μg per injection). siRNA target sequences were for rat (sequence 1) as listed above, under in vitro work. Bridges spanning sciatic transections were processed for immunohistochemistry and probed for NF200 (1:800) and GFAP (1:250). We counted profiles in a line perpendicular to the direction of the bridge in serial fields distally in high-power fields every 270 μm until reaching the last field expressing the heavy-chain neurofilament protein, NF200 (neurofilament; n =3 per group). Counts were made with the observer blinded to the treatment group [25] . For longer-term regeneration experiments, mice were anaesthetised using inhaled 2% isoflurane (Abbott Laboratories) administered through a ventilator in a breathing chamber, shaved and a 3-cm incision was made just below the right hip along the sciatic notch. All three branches of the sciatic nerve were crushed using small blunt-tipped needle driver for 20 s. A small square piece of parafilm was then placed under the crushed sciatic nerve to prevent the siRNA preparation from diffusing into surrounding tissues, and a small piece of surgical gel was placed directly under the injury site and directly on top of the injury site. Over a 20-min interval, 10 μl of saline and siRNA (Rb1 or scrambled) solution was applied every 5 min to the crush area through the surgical gel, totalling to 40 μl. siRNA target sequences were for mouse as listed above, under in vitro work. siRNA scrambled or siRNA Rb1 (Qiagen) was mixed with HiPerFect Transfection Reagent (Qiagen) for at least 20 min at room temperature. Saline was then added to the mixture and it was placed on ice until being administered. After each application of the solution, the nerve was covered with parafilm and the wound was covered with gauze. After 20 min of bathing the nerve in siRNA, the wound was closed with a 3-0 vicryl suture. Twenty microlitres of the siRNA solution was then injected transdermally into the hindpaw on the injured side. All animals were given analgesic Buprenorphine Jell-O (0.5 mg kg −1 ) once daily for 3 days post injury, housed individually in the University of Calgary animal Care Facility with normal light and dark cycles and given free access to food and water. For 5 days post injury, the mice were injected with 40 μl of the siRNA solution through the sutures into the nerve injury site, and 20 μl transdermally into the hindpaw under isoflurane induced anaesthesia. For some of the mice ( n =6 scrambled sequence, n =7 Rb siRNA), injured sciatic nerve and ipsilateral L4-L6 DRG were harvested at 7 days and placed in Trizol reagent for qRT–PCR analysis to verify Rb1 knockdown. The remaining mice were used to assess behavioural and electrophysiological recovery of innervation in the hindpaw. As detailed in previous work, we measured the recovery of hindpaw sensitivity to a hindpaw mechanical sensitivity, to thermal sensitivity and hindpaw grip power [35] . Mechanical sensitivity was measured using an automated Von Frey apparatus (dynamic plantar anesthesiometer, UGO Basile). A filament with a progressively increasing force (2 g s −1 ) was applied to the plantar surface of the mice through the wired mesh until a withdrawal reflex. From three separate measurements in each mouse, the mean latency (time to withdraw) and amount of threshold force were calculated. For testing the recovery of thermal sensation, we used a radiant heat source applied individually to the middle of the hindpaw and the mean latency (s) to withdrawal was calculated from three separate measurements in each mouse. Recovery of multifibre motor and sensory conduction in the hindpaw was also assessed as previously described [35] . Recordings were carried out in sciatic–tibial fibres in mice anaesthetised with isofluorane, at a near-nerve subcutaneous temperature of 37 °C, maintained by a thermosensitive heat lamp with supramaximal stimuli were delivered to the sciatic nerve at the notch and knee. Conduction velocities were calculated in motor axons between the notch and knee and in sensory axons between the knee and paw. Analysis Statistical analysis using one-way ANOVA with Tukey post hoc analysis was performed for qRT–PCR and neurite extension data. When only two experimental groups were compared, a Student’s t -test (paired when appropriate for concurrent data; Welch’s correction for unequal variances and nonparametric tests as appropriate; two-tailed unless otherwise specified; one-tailed when direction of outcome predictable) was used. How to cite this article: Christie, K. J. et al. Enhancing adult nerve regeneration through the knockdown of retinoblastoma protein. Nat. Commun. 5:3670 doi: 10.1038/ncomms4670 (2014).